ARGONAUTE PIWI domain and microRNA duplex structure regulate small RNA sorting inArabidopsis Small RNAs (sRNAs) are loaded into ARGONAUTE (AGO) proteins to induce gene silencing. In plants, the 5′-terminal nucleotide is important for sRNA sorting into different AGOs. Here we show that microRNA (miRNA) duplex structure also contributes to miRNA sorting. Base pairing at the 15th nucleotide of a miRNA duplex is important for miRNA sorting in both Arabidopsis AGO1 and AGO2. AGO2 favours miRNA duplexes with no middle mismatches, whereas AGO1 tolerates, or prefers, duplexes with central mismatches. AGO structure modelling and mutational analyses reveal that the QF-V motif within the conserved PIWI domain contributes to recognition of base pairing at the 15th nucleotide of a duplex, while the DDDE catalytic core of AtAGO2 is important for recognition of the central nucleotides. Finally, we rescued the adaxialized phenotype of ago1-12 , which is largely due to miR165 loss-of-function, by changing miR165 duplex structure which we predict redirects it to AGO2. RNA silencing is a conserved regulatory mechanism mediated by small RNAs (sRNAs) in most eukaryotic organisms [1] , [2] . sRNAs are generated by Dicer (DCR) or DCR-like proteins and then sorted into distinct ARGONAUTES (AGOs), the core components of the RNA-induced silencing complex, to induce silencing of target RNAs or DNAs with complementary sequences. sRNA-based silencing can occur through transcriptional gene silencing by guiding DNA methylation or histone modification, or through post-transcriptional gene silencing by direct cleavage (slicing), destabilization or translational inhibition of target transcripts [2] , [3] . A typical AGO protein consists of four functional domains—N, PAZ, MID and PIWI [4] , [5] —which form a groove structure with the PAZ domain on the top and a crescent structure formed by the MID, PIWI and N domains at the bottom [6] , [7] , [8] . The MID–PIWI interface houses a binding pocket for the 5′ end of the functional guide strand of the sRNA duplex [9] . The PAZ domain contains a binding pocket for the 3′ end of the guide strand, and the PIWI domain harbours a conserved Asp–Asp–His (DDH)/Asp–Asp–Asp (DDD) catalytic core that cleaves the passenger strand of the duplex between nucleotides 10 and 11 of the sRNAs [4] , [10] . The crystal structure of budding yeast Kluyveromyces polysporus AGO shows that an invariant glutamic acid (E) residue is inserted into the catalytic pocket to form the conserved DDHE/DDDE catalytic tetrad for slicing [11] . Studies on AGO structures have focused mainly on yeasts, animals or humans [7] , [8] , [12] , [13] ; so far, the structures of plant AGO proteins are still enigmatic. sRNA sorting into the appropriate AGO is a key step that determines the function of a sRNA. AGOs from different organisms exhibit distinct, yet overlapping, sorting mechanisms. In animals, sRNA sorting is determined by the thermodynamic stability of the duplex termini, the specific protein–protein interactions between the AGO and the DCR complexes, the structure of the sRNA duplex, the sRNA 5′-terminal nucleotide (nt) and the complementarity of the sRNA to its target [14] , [15] , [16] , [17] , [18] . The strand with less stability at its 5′ terminus is incorporated as the guide strand, while the other strand (called the passenger or star strand) is degraded [14] , [15] . In Drosophila melanogaster , miRNA guide strand/miRNA star strand duplexes (miRNA/miRNA*) are generated by the DCR1/Loquacious complex and are subsequently sorted into AGO1 (DmAGO1), whereas siRNA duplexes are processed by the DCR2/R2D2 complex and are sorted into AGO2 (DmAGO2) [16] , [19] . miRNA/miRNA* duplexes often contain central mismatches at nucleotide positions 8–12, whereas siRNA duplexes have perfect or near-perfect complementary sequences. In general, DmAGO1 shows a bias for a 5′-terminal (5′) U, whereas DmAGO2 favours a 5′C (refs 20 , 21 , 22 ). Sequence complementarity between targets and sRNAs also affect sRNA stability and sorting [18] , [23] , [24] . Although sRNA sorting is not well-understood in Caenorhabditis elegans , miRNA duplexes with central mismatches are preferentially sorted into two AGO proteins, Argonaute Like Gene-1 (CeALG-1) and CeALG-2, while siRNA duplexes with perfect base pairing are mainly sorted into another AGO protein, RNA interference-Defective 1 (RDE-1; ref. 25 ). Human AGO2 (HsAGO2) contains a rigid loop in the MID domain that preferentially recognizes 5′U’s or A’s, which reduces the binding efficiency of sRNAs with a 5′C or G (ref. 26 ). Interestingly, this nucleotide specificity loop is conserved in all four HsAGOs. They also have similar sorting preferences for duplexes with central mismatches, which suggests that animal AGOs may not have a strict sorting systems or their sorting mechanism is still not fully understood [27] , [28] . In plants, the 5′-terminal nt of sRNAs is more critical for sRNA sorting into the appropriate AGO than in animals [29] , [30] . Arabidopsis AGO1 (AtAGO1) prefers 21-nt sRNAs with a 5′U, AtAGO2 favours 21-nt sRNAs with a 5′A, AtAGO5 has a bias towards sRNAs with a 5′C but without an obvious size preference, and AtAGO4 preferentially loads 24-nt sRNAs with a 5′A (refs 31 , 32 ). However, the 5′-terminal nt-directed sorting model is not the only mechanism for sRNA sorting in plants. For example, some sRNAs sorted into AtAGO2 do not have a 5′A, such as miR396*, miR165*, miR398*, miR166* and miR156*, while some sRNAs containing a 5′A are sorted into AGOs other than AtAGO2 and AtAGO4, such as miR172 and miR783 (sorted into AtAGO1) or miR390 (sorted into AtAGO7). Some sRNAs containing a 5′C, such as miR169 and miR395, are sorted into AtAGO1. Additional mechanisms for sRNA sorting in plants are still largely unknown, although the importance of sRNA duplex structures has recently been recognized. For example, the specific sorting of miR166 and miR390 into Arabidopsis AtAGO10 and AtAGO7, respectively, is determined by the secondary structure of the miRNA/miRNA* duplex and by the identity of the 5′-terminal nt of the miRNA [33] , [34] . Moreover, miR408 that possesses a 5′A is sorted into both AtAGO1 and AtAGO2 to co-regulate the expression of Plantacyanin [35] . Our previous study has shown that AtAGO2 plays an important role in antibacterial defence through its association with miR393* (ref. 36 ). MiR393* and miR393 originate from the same miRNA duplex and are selectively sorted into AtAGO2 and AtAGO1, respectively. Although the differential sorting of miRNA and miRNA* of the same duplex into different AGOs has been observed in multiple plant and animal species, little is known about the specific features of the miRNAs and/or the AGOs that dictate miRNA strand selection and sorting into the appropriate AGO [21] , [22] , [30] , [37] . In this study, we unveil the important roles of both the secondary structure of miRNA duplexes and the AGO PIWI domain in miRNA sorting in Arabidopsis . We have found that base pairing at the 15th position (#15) of the miRNA duplex is essential for effective sorting into both AtAGO1 and AtAGO2. AtAGO2 favours miRNA duplexes without a mismatch at #11, whereas AtAGO1 tolerates or prefers miRNA duplexes with central mismatches. Structure modelling and mutational analyses of AGO proteins identify the conserved Gln–Phe–Val (QF-V) motif and the catalytic tetrad within the PIWI domain, which contribute to the recognition of nucleotides at #15 and #11 of the miRNA duplex. Finally, the stable expression of an AtAGO2-favoured artificial miR165 duplex with no mismatch at #15 and #11 suppresses the adaxialized phenotype of the ago1-12 mutant that largely resembles the miR165 loss-of-function phenotype. Base pairing at #15 and #11 is essential for AtAGO2 sorting To investigate the impact of the sRNA duplex structure in sRNA sorting into Arabidopsis AGOs, we examined the sorting of miRNA/miRNA*s derived from several duplexes containing mismatches at different positions. These artificial duplexes were modified by altering only the sequence of the passenger strand not containing the miRNA or miRNA* whose sorting was analyzed. Our primary focus was to study miRNA/miRNA*s that are sorted into AtAGO2. We first chose to analyze miR396*, because its duplex has the fewest number of mismatches compared with other duplexes that originate miRNAs associating with AGO2 ( Fig. 1a ) and also generates one of the most abundant sRNAs sorted into AtAGO2. We generated a series of miR396/miR396* duplexes with a mismatch from nucleotides #1–#19 of miR396* by only changing the miR396 nucleotides ( Fig. 1a ). In all cases, the original wobble mismatch at #18 was retained, and the 5′G was replaced by an A to meet the 5′A preference of AtAGO2. Each of these miRNA duplexes was separately co-expressed in Nicotiana benthamiana leaves together with an AtAGO2 protein tagged at its N-terminal region with three tandem repeats of the haemaglutinin (HA) epitope. MiR396* association with AtAGO2 was assessed by co-immunoprecipitation (Co-IP) with HA antibody followed by sRNA Northern blot analysis. As shown in Fig. 1b , a mismatch at #1, #11 or #15 of the miR396/miR396* duplex had the strongest effect on reducing miR396* sorting efficiency into AtAGO2. A mismatch at nucleotides #10 or #19 also reduced miR396* sorting, although to a lesser extent. As nucleotides #1 and #19 are terminal nucleotides of the miRNA duplex, their mismatches would likely interrupt terminal binding in the AGO binding pockets. Thus, we mainly focused on nucleotides #15 and #11 of the miRNA duplex for further characterization. 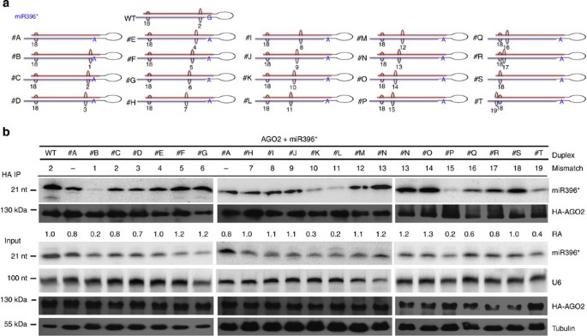Figure 1: Changes in miR396* duplex structure affect miR396* sorting efficiency into AtAGO2. (a) Distinct miR396* duplexes with mismatches at different positions. Red strand: miRNA, purple strand: miRNA*, large bulge: mismatch, small bulge: wobble mismatch, black number: mismatch or wobble position, blue letter: 5′ first nt. (b) miR396* duplexes shown inawere co-expressed with HA–AtAGO2 inN. benthamiana. miR396* was detected from HA–AtAGO2 immunoprecipitated (HA-IP) and input fractions with a miR396* antisense probe. Accumulation of HA–AGO2 in immunoprecipitated (HA-IP) and input fractions is shown in the corresponding Western blots. U6 and tubulin were used as RNA and protein loading controls, respectively. Uncropped images are shown inSupplementary Fig. 13. Relative abundance (RA) indicates the relative fold change of miR396* in each lane compared with immunoprecipitated miR396*WT. These values were assessed with ImageQuant software for each lane by first normalizing the miR396* input levels to U6, then normalizing the immunoprecipitated miR396* levels to those values. Similar results were obtained from more than three biological repeats. Figure 1: Changes in miR396* duplex structure affect miR396* sorting efficiency into AtAGO2. ( a ) Distinct miR396* duplexes with mismatches at different positions. Red strand: miRNA, purple strand: miRNA*, large bulge: mismatch, small bulge: wobble mismatch, black number: mismatch or wobble position, blue letter: 5′ first nt. ( b ) miR396* duplexes shown in a were co-expressed with HA–AtAGO2 in N. benthamiana . miR396* was detected from HA–AtAGO2 immunoprecipitated (HA-IP) and input fractions with a miR396* antisense probe. Accumulation of HA–AGO2 in immunoprecipitated (HA-IP) and input fractions is shown in the corresponding Western blots. U6 and tubulin were used as RNA and protein loading controls, respectively. Uncropped images are shown in Supplementary Fig. 13 . Relative abundance (RA) indicates the relative fold change of miR396* in each lane compared with immunoprecipitated miR396*WT. These values were assessed with ImageQuant software for each lane by first normalizing the miR396* input levels to U6, then normalizing the immunoprecipitated miR396* levels to those values. Similar results were obtained from more than three biological repeats. Full size image We next examined the importance of base pairing at nucleotides #15 and #11 for AtAGO2 sorting of two additional AtAGO2-associated miRNA/miRNA*s, miR393* and miR390. The wild-type miR393*/miR393 duplex has a wobble mismatch at #12 and a gap between #3 and #4 (refs 30 , 36 ). We generated several miR393/miR393* duplexes that retained the wobble mismatch, but lacked the gap, and included a mismatch at #11 or #15 ( Fig. 2a ). As shown in Fig. 2b , a mismatch at #15 or #11 also largely decreased the sorting efficiency of miR393* into AtAGO2. MiR390 is mainly sorted into AtAGO7 (refs 29 , 30 ). It has a 5′A, and associates with AtAGO2 as well. MiR390/miR390* wild-type duplex has a mismatch at #11 ( Fig. 2c ). When we altered the miR390* sequence to remove this mismatch, we observed a noticeable increase in miR390 sorting into AtAGO2 ( Fig. 2d , right panel). When a mismatch at #15 was added by introducing a point mutation in miR390*, miR390 sorting efficiency significantly decreased ( Fig. 2d , left panel). 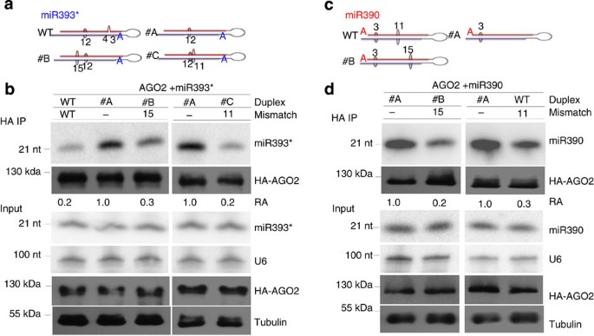Figure 2: Mismatches at #15 and #11 in the miRNA duplex reduce sorting efficiency of miRNAs into AtAGO2. Structures of miR393 and miR390 duplexes with or without a mismatch at #15 or #11 are shown inaandc, respectively, as red strands (miRNAs), purple strands (miRNA*s), bigger bulges (mismatches) and small bulges (wobble pairings).banddmiRNAs were co-expressed with HA–AtAGO2 inN. benthamiana. RNA recovered from HA–AtAGO2 immunoprecipitated (HA-IP) and input fractions were probed to detect specific miRNAs by Northern blot. Accumulation of HA–AGO2 was detected by Western blot. U6 and tubulin were used as controls for RNA and protein blots, respectively. Similar results were obtained from three biological repeats. Uncropped images are shown inSupplementary Fig. 13. Figure 2: Mismatches at #15 and #11 in the miRNA duplex reduce sorting efficiency of miRNAs into AtAGO2. Structures of miR393 and miR390 duplexes with or without a mismatch at #15 or #11 are shown in a and c , respectively, as red strands (miRNAs), purple strands (miRNA*s), bigger bulges (mismatches) and small bulges (wobble pairings). b and d miRNAs were co-expressed with HA–AtAGO2 in N. benthamiana . RNA recovered from HA–AtAGO2 immunoprecipitated (HA-IP) and input fractions were probed to detect specific miRNAs by Northern blot. Accumulation of HA–AGO2 was detected by Western blot. U6 and tubulin were used as controls for RNA and protein blots, respectively. Similar results were obtained from three biological repeats. Uncropped images are shown in Supplementary Fig. 13 . Full size image We also investigated the contribution of miRNA duplex structure on AtAGO2 sorting for miRNAs with a 5′U. First, as shown in Supplementary Fig. 1 , the sorting efficiency of both miR165-5′U and miR165-5′A originated from duplexes containing mismatches at #15 is lower than that of the corresponding miRNAs originated from duplexes without #15 mismatches. And second, a mismatch at #11 of the miRNA duplex reduced the sorting into AtAGO2 of both 5′U and 5′A versions of miR396* and miR165 ( Supplementary Fig. 2 ). Therefore, in addition to confirming that a 5′A facilitates miRNA sorting into AtAGO2, these results show that mismatches at #11 and #15 of the miRNA duplex also reduce the sorting of miRNA or miRNA*s with a 5′U into AtAGO2. Taken together, these results indicate that, in addition to the known 5′-terminal nt identity sorting rule, base pairing at #15 and #11 of the miRNA duplex is also critical for effective miRNA sorting into AtAGO2. A #15- but not #11-mismatch interferes with AtAGO1 sorting We then tested whether the base pairing requirements at #15 and #11 of the miRNA duplex for AtAGO2 sorting was also valid for AtAGO1, the major miRNA-binding AGO in Arabidopsis . The miR165/miR165* duplex was studied because miR165 is one of the most abundant miRNAs associated with AtAGO1. The miR165 duplex has a rather complex structure with four mismatches (at #5, #12, #13 and #17) and two wobble mismatches (at #4 and #10). An extra mismatch at #15 was introduced by mutating the miR165* sequence ( Fig. 3a ), which largely reduced miR165 sorting into AtAGO1 ( Fig. 3b , left panel). To test the effect of the mismatch at #11 in AtAGO1 sorting, we first removed mismatches at #12 and #13 and the wobble at #10 to make the central region clear of mismatches. Then, we introduced a mismatch at #9, #10 or #11 ( Fig. 3a ). We found that AtAGO1 tolerated or even favoured central mismatches ( Fig. 3b , right panel). Similar results were observed when testing AtAGO1 binding of miR162, another AtAGO1-associated miRNA with fewer mismatches in its duplex. Adding a mismatch at #15 also largely reduced miR162 sorting into AtAGO1 ( Fig. 3c,d left panel), suggesting that base pairing at #15 is important for miRNA sorting into both AtAGO1 and AtAGO2. The wild-type miR162 duplex contains a mismatch at #11. MiRNA sorting into AtAGO1 was almost the same when the mismatch at #11 was removed from the miR162/miR162* duplex ( Fig. 3c,d right panel), supporting the conclusion that, unlike AtAGO2, AtAGO1 tolerates a central mismatch in the miRNA duplex. 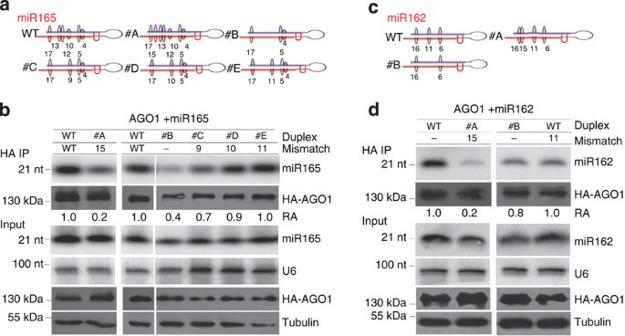Figure 3: Mismatches at #15 and in the central region of miRNA duplexes regulate miRNA sorting efficiency into AtAGO1. Structures of miR165 and miR162 duplexes with mismatches at different positions are shown inaandc, respectively, as red strands (miRNAs), purple strands (miRNA*s), bigger bulges (mismatches) and small bulges (wobble pairings).banddThe miRNA duplexes were co-expressed with HA–AtAGO1 inN. benthamiana.RNA recovered from HA–AtAGO1 immunoprecipitated (HA-IP) and input fractions were probed to detect specific miRNAs by Northern blot. Accumulation of HA–AGO1 was detected by Western blot using HA antibody. U6 and tubulin were used as controls for RNA and protein blots, respectively. Similar results were observed in more than two biological repeats. Uncropped images are shown inSupplementary Fig. 13. Figure 3: Mismatches at #15 and in the central region of miRNA duplexes regulate miRNA sorting efficiency into AtAGO1. Structures of miR165 and miR162 duplexes with mismatches at different positions are shown in a and c , respectively, as red strands (miRNAs), purple strands (miRNA*s), bigger bulges (mismatches) and small bulges (wobble pairings). b and d The miRNA duplexes were co-expressed with HA–AtAGO1 in N. benthamiana. RNA recovered from HA–AtAGO1 immunoprecipitated (HA-IP) and input fractions were probed to detect specific miRNAs by Northern blot. Accumulation of HA–AGO1 was detected by Western blot using HA antibody. U6 and tubulin were used as controls for RNA and protein blots, respectively. Similar results were observed in more than two biological repeats. Uncropped images are shown in Supplementary Fig. 13 . Full size image We also studied the contribution of miRNA duplex structure on AtAGO1 sorting for miRNAs with a 5′A terminal nt. First, a mismatch at #15 of the miRNA duplex reduced the sorting of both miR165-5′A and miR165-5′U into AtAGO1 ( Supplementary Fig. 3 ). And second, AtAGO1 tolerated or even preferred a mismatch at #11 of miR165-5′U, miR165-5′A, miR396*-5′U and miR396*-5′A ( Supplementary Fig. 4 ). Therefore, both the 5′-terminal nt and the secondary structure of the miRNA/miRNA* clearly contribute to the sorting of miRNA/miRNA*s into AtAGO1. Finally, to further validate the contribution of the miRNA duplex structure on the sorting of miRNAs into AtAGOs, we analyzed published high throughput sequencing data sets from untreated Arabidopsis , including AtAGO1- and AtAGO2-associated sRNAs [24] . Out of the 15 miRNAs or miRNA*s that are at least twofold enriched in AtAGO2 IP fraction compared with the input sample (total RNA), only one (6.6%) was derived from miRNA duplexes containing a mismatch at #15 ( Supplementary Data 1a ). Similarly, in AtAGO1 IP fraction, only one out of the 35 (2.9%) enriched miRNAs or miRNA*s was derived from duplexes containing a mismatch at #15 ( Supplementary Data 1b ). On the other hand, 12 out of the 15 (80.0%) miRNAs or miRNA*s enriched in AtAGO2 IP fraction were derived from duplexes with no central mismatches (#9–#12) ( Supplementary Data 1a ), whereas 23 out of the 35 (65.7%) miRNAs or miRNA*s enriched in AtAGO1 IP fraction originated from duplexes with central mismatches ( Supplementary Data 1b ). These data support our experimental results that (i) base pairing at #15 is essential for sRNA sorting into both AtAGO1 and AtAGO2, and (ii) AtAGO2 favours sRNA duplexes with no central mismatches, whereas AtAGO1 can tolerate central mismatches. The QF-V motif contributes to the recognition of #15 pairing We hypothesized that recognition of the miRNA duplex structure is determined by certain motifs in AGO proteins. The identification of the specific amino acid residues that recognize these miRNA duplex structures could help us better understand the sorting mechanisms of miRNAs into specific plant AGOs. Although the crystal structure of a plant AGO is yet to be resolved, the crystal structure of HsAGO was recently described [7] , [8] , [12] , [13] . The AtAGO2 structure was modelled with a miR396* duplex ( Fig. 4a ) based on the HsAGO structure, from which the function of some residues and motifs have been revealed. 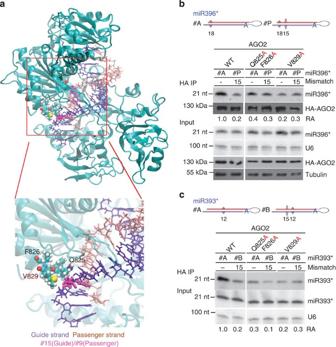Figure 4: The QF-V residues of AtAGO2 PIWI domain contribute to its bias for miRNAs derived from duplexes without mismatches at #15. (a) A stereo view of the interaction between AtAGO2 and the miRNA guide strand (purple) and passenger strand (grey) at #15 of the miRNA duplex. Inset box is enlarged to show residues in the PIWI domain located near #15. The Mid (top), PIWI (middle) and N (bottom) domains are shown on the left, and the PAZ domain is presented on the right. The labelled residues represent QF-V amino acids that potentially recognize the nucleotide at #15 (pink). miR396/miR396* (b) and miR393/miR393* (c) duplexes with or without mismatches at #15 were co-expressed with HA–AtAGO2 QF-V mutants inN. benthamiana. Duplexes are shown with red strands (miRNAs), purple strands (miRNA*s), bigger bulges (mismatches) and small bulges (wobble pairings). miRNA recovered from HA–AtAGO2 immunoprecipitated (HA-IP) and input fractions were detected by Northern blot. Accumulation of HA–AGO2 was detected by Western blot using HA antibody. U6 and tubulin were used as controls for RNA and protein blots, respectively. Similar results were obtained from three biological repeats. Uncropped images are shown inSupplementary Fig. 13. Figure 4: The QF-V residues of AtAGO2 PIWI domain contribute to its bias for miRNAs derived from duplexes without mismatches at #15. ( a ) A stereo view of the interaction between AtAGO2 and the miRNA guide strand (purple) and passenger strand (grey) at #15 of the miRNA duplex. Inset box is enlarged to show residues in the PIWI domain located near #15. The Mid (top), PIWI (middle) and N (bottom) domains are shown on the left, and the PAZ domain is presented on the right. The labelled residues represent QF-V amino acids that potentially recognize the nucleotide at #15 (pink). miR396/miR396* ( b ) and miR393/miR393* ( c ) duplexes with or without mismatches at #15 were co-expressed with HA–AtAGO2 QF-V mutants in N. benthamiana . Duplexes are shown with red strands (miRNAs), purple strands (miRNA*s), bigger bulges (mismatches) and small bulges (wobble pairings). miRNA recovered from HA–AtAGO2 immunoprecipitated (HA-IP) and input fractions were detected by Northern blot. Accumulation of HA–AGO2 was detected by Western blot using HA antibody. U6 and tubulin were used as controls for RNA and protein blots, respectively. Similar results were obtained from three biological repeats. Uncropped images are shown in Supplementary Fig. 13 . Full size image Our AtAGO2 model shows that the nucleotide at #15 of the miRNA duplex resides close to Q825, F826 and V829 within the PIWI domain of AtAGO2 ( Fig. 4a ). The Q residue is conserved in all plant and animal AGOs we examined, and the F residue is also conserved in all plant and animal AGOs except for HsAGO1, which has a similar hydrophobic leucine (L) residue instead. The V residue is conserved in all plant AGOs and most animal AGOs except for HsAGO1 and DmAGO2, in which the V is replaced by a similar isoleucine (I) residue ( Supplementary Fig. 5 ). The highly conserved nature of QF-V motif across different kingdoms suggests their critical role in the function of AGOs. Because molecular modelling is a prediction and may substantially differ from its real structure, further validation by mutational analysis and future AtAGO2 crystallization analysis is necessary. To test whether these residues are important for recognition of nucleotide base pairing at #15, two constructs were made, AtAGO2-Q825A/F826A and AtAGO2-V829A, in which residues Q825, F826 and V829 were mutated to an alanine (A). Importantly, these mutations did not affect the stability of the AtAGO2 protein variants ( Supplementary Fig. 6a ). As shown in Fig. 4b,c , a single mutation of V829A or a double mutation of Q825A/F826A reduced the sorting of miR396* and miR393*, which were derived from duplexes lacking a mismatch at #15, into AtAGO2. However, the sorting efficiency of sRNAs derived from duplexes with a mismatch at #15 did not change. This result suggests that AtAGO2 variants carrying mutations in the QF-V motif lost their preference for #15 base pairing ( Fig. 4b,c ). Thus, the QF-V motif within the PIWI domain is involved in AtAGO2 preferential sorting of miRNA duplexes without a mismatch at #15. To test whether this conserved QF-V motif is also important for AtAGO1 sorting, we introduced the same series of point mutations into AtAGO1. All mutated versions of AtAGO1 accumulated to a similar level as wild-type AtAGO1 ( Supplementary Fig. 6b ). Similarly, the sorting preference for miR165 derived from a duplex without a #15 mismatch was lost in AtAGO1-V858A and AtAGO1-Q854A/F855A mutants, whereas the sorting efficiency of a miR165 derived from a duplex with a #15 mismatch was not affected ( Supplementary Fig. 7 ). Taken together, these results suggest that the QF-V motif in both AtAGO1 and AtAGO2 contributes to the recognition of #15 base pairing within sRNA duplexes. The catalytic tetrad contributes to the recognition of #11 AtAGO2 prefers miRNAs originating from duplexes without a mismatch at #11, whereas AtAGO1 tolerates or even prefers duplexes with central mismatches. The AtAGO2 model shows that the nucleotide at #11 is located near the DDDE catalytic tetrad of AtAGO2 ( Fig. 5a , left panel). AtAGO2 and AtAGO3 are the only AtAGOs that contain a DDDE motif, while AtAGO1 and other AtAGOs encode a conventional DDHE motif ( Supplementary Fig. 5 ). To determine the role of the catalytic domain on central mismatch selection bias, we tested the AtAGO2-DDD954H and AtAGO1-DDH988D forms in which the third residue of the AtAGO2 DDD and the AtAGO1 DDH was swapped. These mutations did not interfere with AGO protein accumulation ( Supplementary Fig. 6 ) as reported previously [38] . The sorting bias of wild-type AtAGO2 and the AtAGO2-DDD954H mutant was examined by testing their association with miR396* derived from miRNA duplexes without (#A) or with (#L) a central mismatch ( Fig. 5b ). As predicted, the AtAGO2-D954H mutant was no longer able to discriminate against duplex #L that carries a mismatch at #11 ( Fig. 5b left panel), suggesting that residue D954 contributes to the sorting preference of duplexes without central mismatches for AtAGO2. Similar results were observed when testing the sorting efficiency of miR393* derived from duplexes with or without a mismatch at #11 ( Fig. 5c left panel). Thus, the catalytic core residue D954 of AtAGO2 contributes to the sorting bias for miRNA duplexes without central mismatches. However, a single amino acid change from H to D in AtAGO1 did not reduce its association with miR165 derived from a duplex with a mismatch at #11 ( Supplementary Fig. 8 ). This result suggests that the catalytic core residue H988 of AtAGO1 has little impact on its miRNA sorting efficiency, and the conversion to a D residue did not confer AtAGO1 the ability to select against duplexes without central mismatches, which may also require other residues. 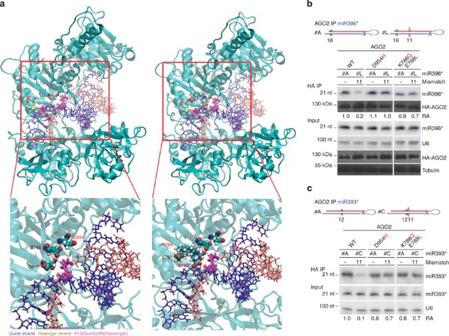Figure 5: The catalytic domain and the KEE motif determine the AtAGO2 sorting bias. (a) The stereo views (top panel) and enlarged detailed views of the interaction between AtAGO2 protein (cyan) with the guide strand (blue) and passenger strand (grey). Structures of AtAGO2 displaying DDD (left) and AtAGO2 KEE (right) were predicted by homology modelling. The selected DDD catalytic domain and KEE motif are shown as coloured atoms. Nucleotides #11 of the guide strand and #9 of the passenger strand are indicated in pink. miR396/miR396* (b) and miR393/miR393* (c) duplexes with varying mismatches were co-expressed with HA–AtAGO2 inN. benthamiana. Duplexes are shown as red strands (miRNAs), purple strands (miRNA*s), bigger bulges (mismatches) and small bulges (wobble pairings). miRNA recovered from HA–AtAGO2 immunoprecipitated (HA-IP) and input fractions were detected by Northern blot. Accumulation of HA–AGO2 was detected by Western blot using HA antibody. U6 and tubulin were used as controls for RNA and protein blots, respectively. Similar results were obtained from three biological repeats. Uncropped images are shown inSupplementary Fig. 13. Figure 5: The catalytic domain and the KEE motif determine the AtAGO2 sorting bias. ( a ) The stereo views (top panel) and enlarged detailed views of the interaction between AtAGO2 protein (cyan) with the guide strand (blue) and passenger strand (grey). Structures of AtAGO2 displaying DDD (left) and AtAGO2 KEE (right) were predicted by homology modelling. The selected DDD catalytic domain and KEE motif are shown as coloured atoms. Nucleotides #11 of the guide strand and #9 of the passenger strand are indicated in pink. miR396/miR396* ( b ) and miR393/miR393* ( c ) duplexes with varying mismatches were co-expressed with HA–AtAGO2 in N. benthamiana . Duplexes are shown as red strands (miRNAs), purple strands (miRNA*s), bigger bulges (mismatches) and small bulges (wobble pairings). miRNA recovered from HA–AtAGO2 immunoprecipitated (HA-IP) and input fractions were detected by Northern blot. Accumulation of HA–AGO2 was detected by Western blot using HA antibody. U6 and tubulin were used as controls for RNA and protein blots, respectively. Similar results were obtained from three biological repeats. Uncropped images are shown in Supplementary Fig. 13 . Full size image As shown in Fig. 5a (right panel), the E residue of the DDDE catalytic core forms a Lys–Glu–Glu (KEE) motif and is also located near #11 of the miRNA duplex. The central E787 of AtAGO2 is conserved in all AGOs, but the adjacent residues K786 and E788 are not ( Supplementary Fig. 5 ). This adjacent E is only present in AtAGO2, AtAGO3 and DmAGO2, while AtAGO1 contains an adjacent L, and all the other AtAGOs encode a L or a similar amino acid (I or methionine (M)) [11] . The adjacent residue ‘I’ was present in DmAGO1, CeALG-1, HsAGO1, HsAGO2, HsAGO3 and HsAGO4 ( Supplementary Fig. 5 ), all of which prefer duplexes with central mismatches, while AtAGO2 and DmAGO2 with an adjacent E residue discriminate against duplexes with central mismatches. Therefore, we hypothesized that this motif might also contribute to the sorting bias of AtAGO2 and AtAGO1 for central mismatches. To test this hypothesis, we generated an AtAGO2 mutant by swapping its KEE motif with the AtAGO1 QEL motif. The AtAGO2-K786Q-E-E788L mutant lost its ability to distinguish the difference between duplexes with or without central mismatches, and it showed a similar sorting efficiency for miR396* and miR393* derived from duplexes with or without a mismatch at #11 ( Fig. 5b,c ). This result suggests that the KEE motif is also important for AtAGO2 to recognize the central region of the miRNA duplex structure. However, AtAGO1-Q802K-E-L804E did not associate more efficiently with miR165 derived from duplexes without a central mismatch compared with AtAGO1-WT ( Supplementary Fig. 8 ). Taken together, our results show that both D954 and the KEE motif within the PIWI domain of AtAGO2 are important, but not sufficient, for the selective sorting of miRNAs derived from duplexes without central mismatches. Suppression of ago1-12 by altering miR165 duplex structure Given that different AGOs preferentially load miRNAs from duplexes with different secondary structures, it may be possible to direct a miRNA into a specific AGO by redesigning the miRNA duplex secondary structure through modification of the passenger strand sequence. To test this possibility and to validate our findings demonstrated above, we designed a series of miR165-based duplexes to confirm the favoured duplex structure for AtAGO2. Because AtAGO2 preferentially associates with miRNAs with a 5′A (refs 29 , 30 ), we changed the 5′U of miR165 to an A in all of the constructs expressing different miR165 duplex configurations. As predicted, adding a mismatch in #15 (#G duplex) largely reduced miR165 sorting into AtAGO2 in a N. benthamiana transient assay ( Fig. 6a,b ). To test the effect of central mismatches in miRNA sorting, we first removed the mismatches in the central regions, including those at #12 and #13 as well as the wobble mismatch at #10. Mismatches at the central region (#10, #11 and #12) also clearly reduced sorting of miR165 into AtAGO2 ( Fig. 6a,b ). Furthermore, duplex configuration ‘M’, in which all the mismatches between #4 and #17 were removed and only the mismatches at #4 and #17 were maintained, had the highest sorting efficiency into AtAGO2 ( Fig. 6a,b ). To test whether the miR165 generated from the duplex ‘M’ is functional, miR165 target PHABULOSA (PHB) was co-expressed in N. benthamiana with the miR165 duplex ‘M’ and AtAGO2. As shown in Fig. 6c,d , the accumulation of both PHB messenger RNA (mRNA) and protein was significantly reduced when co-expressed with the miR165 duplex ‘M’ than with the miR165 duplex ‘J’, which contains a mismatch at #11. Thus, the miR165 generated from the duplex ‘M’ configuration is functional in vivo . 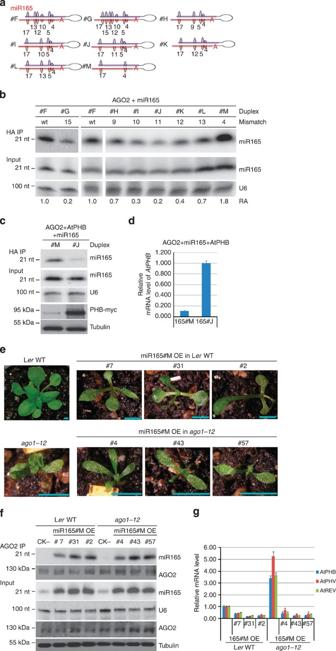Figure 6: An artificial miR165 designed to be sorted into AtAGO2 is functionalin vivo. (a) Structures of miR165 duplexes with mismatches at different positions with red strands (miRNAs), purple strands (miRNA*s), bigger bulges (mismatches) and small bulges (wobble pairings). (b) The miR165M duplex has the highest sorting efficiency with AtAGO2 from theN. benthamianatransient expression assay. Mismatches at central positions or at #15 of miR165 duplex decreased the sorting efficiency of miR165 into AtAGO2. miR165 recovered from HA–AtAGO2 immunoprecipitated (HA-IP) and input fractions was detected by Northern blot. Similar results were obtained from three biological repeats. (c) miR165 derived from the miR165M duplex is predicted to function through association with AtAGO2 when AtAGO2 was co-expressed with miR165 and 35S-PHB-myc inN. benthamiana. The PHB-myc protein was detected by Western blot using myc antibody. Tubulin was used as a loading control. Similar results were obtained from four biological repeats. (d) PHB mRNAs were coordinately downregulated when co-expressed with AtAGO2 and miR165. The expression of PHB genes incwas analyzed by quantitative real-time PCR. Error bars represent s.d. from three technical repeats.N. benthamianaubiquitin was used as an internal control. Similar results were obtained from three biological repeats. (e) TransgenicArabidopsisplants overexpressing the miR165M duplex suppressed the adaxialized phenotype ofago1-12(scale bars, 5 mm). Transgenic miR165M plants were generated in both Lerwild-type (WT) andago1-12backgrounds. Plants were grown under 12-h light, and pictures were taken of 4-week-old plants. (f) Transgenic miR165M plants with high accumulation of miR165 in LerWT andago1-12plants were selected. U6 and tubulin were used as controls for RNA and protein blots, respectively. Similar results were obtained from two generations. (g) miR165 target RNAs—PHB/PHV/REV—were downregulated in miR165M overexpression (OE) plants.AtActin2was used as an internal control for quantitative real-time PCR. Error bars represent s.d. from three technical repeats. Similar results were obtained from three biological repeats. Uncropped images are shown inSupplementary Fig. 13. Figure 6: An artificial miR165 designed to be sorted into AtAGO2 is functional in vivo . ( a ) Structures of miR165 duplexes with mismatches at different positions with red strands (miRNAs), purple strands (miRNA*s), bigger bulges (mismatches) and small bulges (wobble pairings). ( b ) The miR165M duplex has the highest sorting efficiency with AtAGO2 from the N. benthamiana transient expression assay. Mismatches at central positions or at #15 of miR165 duplex decreased the sorting efficiency of miR165 into AtAGO2. miR165 recovered from HA–AtAGO2 immunoprecipitated (HA-IP) and input fractions was detected by Northern blot. Similar results were obtained from three biological repeats. ( c ) miR165 derived from the miR165M duplex is predicted to function through association with AtAGO2 when AtAGO2 was co-expressed with miR165 and 35S-PHB-myc in N. benthamiana . The PHB-myc protein was detected by Western blot using myc antibody. Tubulin was used as a loading control. Similar results were obtained from four biological repeats. ( d ) PHB mRNAs were coordinately downregulated when co-expressed with AtAGO2 and miR165. The expression of PHB genes in c was analyzed by quantitative real-time PCR. Error bars represent s.d. from three technical repeats. N. benthamiana ubiquitin was used as an internal control. Similar results were obtained from three biological repeats. ( e ) Transgenic Arabidopsis plants overexpressing the miR165M duplex suppressed the adaxialized phenotype of ago1-12 (scale bars, 5 mm). Transgenic miR165M plants were generated in both L er wild-type (WT) and ago1-12 backgrounds. Plants were grown under 12-h light, and pictures were taken of 4-week-old plants. ( f ) Transgenic miR165M plants with high accumulation of miR165 in L er WT and ago1-12 plants were selected. U6 and tubulin were used as controls for RNA and protein blots, respectively. Similar results were obtained from two generations. ( g ) miR165 target RNAs—PHB/PHV/REV—were downregulated in miR165M overexpression (OE) plants. AtActin2 was used as an internal control for quantitative real-time PCR. Error bars represent s.d. from three technical repeats. Similar results were obtained from three biological repeats. Uncropped images are shown in Supplementary Fig. 13 . Full size image The Arabidopsis ago1-12 mutant (L er background) carries the H765L mutation in the PIWI domain that lies near the nucleotide at #11 of the miRNA duplex ( Supplementary Figs 5 and 9 ). Similar to what was described for the H977 residue in an AGO of K. polysporus , the mutation of H765 to L or A did not disturb miRNA sorting into AtAGO1 but did abolish AtAGO1 mediated silencing of PHB ( Supplementary Fig. 9 ) [5] , [11] . The ago1-12 mutant has adaxialized trumpet-shaped leaves that curl upwards ( Fig. 6e ) [39] , which largely resemble the phenotype of gain-of-function mutant phb-1d or a miR165-resistant PHB overexpression plant [40] , [41] , [42] . This suggests that the phenotype of ago1-12 mutant is largely due to the loss-of-function of miR165, which leads to over-accumulation of its targets—PHB family proteins. If we could redirect sorting of miR165 into AtAGO2 by altering its passenger strand sequences, we would expect that it could suppress the adaxialized phenotype of ago1-12 caused by the loss-of-function of miR165. To this purpose, we generated Arabidopsis transgenic plants overexpressing miR165 from the duplex ‘M’ configuration (miR165M), previously shown to be functional in N. benthamiana ( Fig. 6c,d ), in the ago1-12 mutant as well as in wild-type L er plants. MiR165 accumulation in the miR165M overexpression (miR165M-OE) plants was analyzed in leaves by sRNA Northern blot to identify highly-expressed lines ( Supplementary Fig. 10 ). The miR165M-OE lines in the wild-type background displayed strong abaxialized phenotypes with leaves curling downward or with even pinhead-shaped leaves ( Fig. 6e,f ). Similarly, ago1-12 plants overexpressing the miR165M duplex also displayed an abaxialized phenotype that resembled the wild-type L er overexpression lines ( Fig. 6e,f ). In the leaves from the miR165M-OE lines, miR165 associated with AtAGO2 ( Fig. 6f ), and miR165 target genes ( PHB, PHAVOLUTA (PHV) , and REVOLUTA (REV) ), were downregulated ( Fig. 6g ). To rule out the possibility that miR165M may be sorted into AtAGOs other than AtAGO2 to suppress PHB expression in these miR165M-OE lines, we examined (1) miR165M sorting efficiency in all the nine AtAGOs known to be expressed in Arabidopsis (AtAGO2—AtAGO7 and AtAGO9—AtAGO10; AtAGO8 was not included because it was annotated as a pseudogene), and (2) the accumulation of its target PHB. AGO1-H765L was used as a control. As expected, miR165M was efficiently loaded into AtAGO2, but surprisingly also into AtAGO4, AtAGO6 and AtAGO9, three AGOs known to load 24-nt sRNAs and be involved in RNA-directed DNA methylation pathway ( Supplementary Fig. 11a ). MiR165M was also sorted rather poorly into AtAGO3 and AtAGO7, two AGOs from the same subgroup as AtAGO2 (ref. 36 ; Supplementary Fig. 11a ). A trace amount of miR165 was also found in AtAGO5 and AtAGO10. These AtAGOs were functional in terms of sRNA sorting, as shown by efficient sorting of miR390, miR390* ( Supplementary Fig. 11a ) and miR165WT ( Supplementary Fig. 11b ) into AtAGO7, AtAGO5, and AtAGO1 or AtAGO10, respectively. The accumulation of the miR165M target PHB was also co-expressed and analyzed to evaluate the function of each AtAGO/miR165M complex. PHB protein accumulation was reduced in the presence of AtAGO2, and also in AtAGO3 and AtAGO5 to a lesser degree. However, PHB protein accumulation was not changed when AtAGO4, AtAGO6, AtAGO9, AtAGO7 and AtAGO10 were co-expressed. Note that although AtAGO5 did not associate efficiently with miR165M, PHB accumulation was also slightly reduced when AtAGO5 was co-expressed, most likely due to the sorting of endogenous miR165WT ( Supplementary Fig. 11b ). Efficient sorting of miR165WT into AtAGO4, AtAGO6 and AtAGO10 was also observed ( Supplementary Fig. 11b ), providing additional evidence that neither AtAGO4, AtAGO5, AtAGO6 nor AtAGO10 could rescue the ago1-12 phenotype; otherwise, we would have only seen the ago1-12 phenotype in ago1-12 double mutants with these AGOs. Finally, expression analysis of AtAGO2, AtAGO3 and AtAGO5 mRNAs in different tissues showed that only AtAGO2 mRNA is accumulated in ago1-12 leaves, while AtAGO5 is mainly accumulated in flowers and siliques and AtAGO3 is mostly expressed in roots, flowers and siliques ( Supplementary Fig. 12 ), in agreement with previous microarray data [31] . Taken together, these results strongly support that miR165 generated from miR165M duplexes was functional in vivo through AtAGO2. The sorting of sRNAs into AGO proteins is a key step in RNA silencing pathways. First, we have found that the secondary structure of miRNA duplexes plays a significant role in AGO sorting. miRNAs with the same 5′-terminal nt but derived from different secondary structures were sorted into AtAGOs with different efficiencies. Second, using structure modelling and mutational analysis, we identified functional motifs within the PIWI domain of AGOs that are responsible for structural recognition of the miRNA duplex. A mismatch at #15 in miRNA duplexes reduces miRNA sorting efficiency in both AtAGO2 and AtAGO1. The QF-V motif that resides near the nucleotide at #15 is involved in the recognition of the base pairing at this position. AGOs with mutations at QF or V lost their preference for the base pairing at #15. The Q residue is conserved in all analyzed AGOs from Arabidopsis , humans, Drosophila and Neurospora crassa ( Supplementary Fig. 5 ). The F and V residues are conserved in all Arabidopsis AGOs, as well as in HsAGO2, DmAGO1 and N. crassa QDE2 ( Supplementary Fig. 5 ). Such a high degree of conservation strongly suggests that the QF-V motif is imperative to AGO function. The HsAGO2 structure studies also suggest that this motif may contribute to the binding of sRNA [7] , [8] , supporting its essential role in AGO function. AtAGO2 associates preferentially with miRNAs derived from duplexes without central mismatches, whereas AtAGO1 tolerates or prefers miRNAs derived from duplexes with central mismatches. Although switching the catalytic core residue D954 to H does not appear to change AGO2 slicing activity [38] , our structure modelling and domain swap analysis demonstrated that the DDDE catalytic tetrad within the PIWI domain of AtAGO2 contributes to the sorting preference for miRNAs derived from duplexes without middle mismatches. AGO2 carrying D954H or K786Q-E-E788L mutations lost its preference for duplexes without central mismatches, and could tolerate duplexes with central mismatches. Similarly, DmAGO2 also preferentially binds duplexes without central mismatches, while DmAGO1 has the same preference as AtAGO1, which tolerates or prefers duplexes with central mismatches [16] . DmAGO2 encodes a LEE motif, which is highly similar to the KEE motif in AtAGO2, supporting the importance of this motif in preferential binding of duplexes without central mismatches. The catalytic core DDDE is only present in eukaryotic AtAGO2, AtAGO3 and N. crassa QDE2 and prokaryotic Thermus thermophilus AGO, while DDHE is the most common catalytic core for most AGOs, including DmAGO2. However, AtAGO1 with a H988D mutation or with the KEE motif cannot distinguish between duplexes with or without central mismatches as AtAGO2 does, indicating that these motifs are important but not sufficient to discriminate against duplexes with central mismatches. These results suggest that other amino acids may be required in addition to these residues. Further analysis is required for identification of such peripheral residues or motifs. Furthermore, in addition to AGO proteins, double-stranded RNA-binding proteins, such as DRB1, DRB2, DRB3, DRB4 and DRB5 in Arabidopsis , are believed to contribute to RNA silencing. In the drb1 mutant, most of the miRNAs have decreased abundance and most of the miRNA*s have increased abundance, while in the drb2345 quadruple mutant, the opposite is true [43] . As most miRNAs are sorted into AtAGO1, while many miRNA*s are sorted into AtAGO2, these dsRBPs are also likely to interfere with the sorting of sRNAs into different AtAGOs. A better understanding of AGO sorting mechanisms will benefit both the functional study as well as the application of RNA silencing. Many organisms encode a large number of AGOs, which participate in distinct RNA silencing pathways. They may have evolved different mechanisms for sRNA sorting and function. The 5′-terminal nt and the structure of sRNA duplexes play an important role in AGO sorting. However, there are still several AGO sorting phenomena and RNA silencing functions that cannot be fully explained by the 5′-terminal nt or duplex structure rules. Therefore, further functional studies are required to better elucidate the mechanisms of sRNA sorting in plants. Vector construction The DNA fragments of miRNA precursors pre-miR396a*, pre-miR393b*, pre-miR390a, pre-miR390b, pre-miR165a and pre-miR162 were cloned from genomic DNA with corresponding oligos ( Supplementary Data 2 ). The DNA fragment of amiRNA/amiRNA* was amplified by PCR using synthesized long oligos. These fragments were cloned into pENTR vector and then cloned into destination vector pEarleyGate 100 (pEG100). The genomic DNA fragment of 3HA–AtAGO2 and complementary DNA fragment of 3HA–AtAGO1 were amplified from pMDC32-AGO2/AGO1 (ref. 29 ) and cloned into pENTR vectors. Point mutations in AtAGO1 and AtAGO2 were introduced into pENTR-3HA–AGO1 and pENTR-3HA–AGO2, respectively, using the GENEART Site-Directed Mutagenesis System. These AGO fragments were then cloned into pMDC32. 35S-HAAGO3, 35S-HAAGO4, 35S-HAAGO5, 35S-HAAGO6, 35S-HA AGO7, 35S-HAAGO9, 35S-HAAGO10 and 35S-PHB were previously described [44] , [45] . Plant growth, transient expression and transformation Arabidopsis and N. benthamiana plants were grown at 23 °C in a 12-h light/12-h dark photoperiod. Agrobacterium GV3101 cultures transformed with pEG100-miRNA or pMDC32-AGO were grown overnight at 28 °C with 20 μM acetosyringone. The Agrobacterium containing either AGO or a sRNA duplex was adjusted to a concentration of OD 600 =1.0 and then mixed in equal proportions. Three-week-old N. benthamiana plants were infiltrated with the mixed Agrobacterium . The transient expression tissue was collected 3 days post inoculation. Agrobacterium containing pEG100-miRNAs was incubated similarly and transformed into genotyped ago1-12 +/− plants. IP, RNA analysis and protein analysis RNA IP of HA–AtAGO1/HA–AtAGO2 was performed as previously described [36] . Briefly, 2 g N. benthamiana tissue or 0.5 g Arabidopsis tissue was ground and dissolved in IP extraction buffer. After spinning, the lysates were used for RNA extraction using Trizol for the RNA input and protein extraction for protein input. The same lysates were pre-cleaned with protein A beads (Roche, 11134515001) and then immunoprecipitated with AtAGO2 antibody or HA-beads (Roche, 43400075). The washed beads were then used for RNA and protein analysis. Total RNA (40 μg) was used for input control. Total and immunoprecipitated fractions are probed with HA antibody (Santa cruz, NC9929626), c-myc antibody (Santa cruz, SC-786), and tubulin antibody (Sigma-Aldrich, T6074). The uncropped blots are shown in Supplementary Fig. 13 . Input total RNA (5 μg) was treated with DNase I and then used for reverse transcription and subsequent quantitative real-time PCR. Structure prediction The structure of HmAGO2 (PDB ID 4EI3; refs 7 , 8 ) and HmAGO1 (PDB ID 4KRF; refs 12 , 13 ) were used for the construction of AtAGO1 and AtAGO2 models. First, multiple sequence alignments were performed using VMD software and the T-Coffee program [46] , [47] . Different templates were used to build the initial homology models, and crystal structures 4EI3 (32% sequence identity to AtAGO2) and 4KRF (35% sequence identity to AtAGO1) were selected as the template to build our models based on their sequence identity and the torsion angle energy in the trail models. SWISS-MODEL ( http://swissmodel.expasy.org/ ) Alignment Mode was used for the homology modelling [48] . The double-stranded mir396* RNA structure was built with VMD and VegaZZ programs [49] . The structure was then refined to ensure correct intramolecular contacts. The RNA was then docked to apo AtAGO2 and the energy of the complex was minimized by removing clashes and optimizing intermolecular interactions. All molecular mechanics calculations were performed with CHARMM force field using VMD and NAMD programs [50] , [51] . Survey of sRNA duplex sorted into AGOs The survey was performed with published high throughput sequencing data sets containing AtAGO1- and AtAGO2-sorted sRNAs [30] . A two-time enrichment was set as the cut-off. The small RNAs generated from the different loci but containing the same structure and sequence were counted as 1 (for example, miR166a, miR166b and miR166c in AtAGO1 data set). The miR159b in AtAGO2 was not counted as the linker bias due to its un-methylated ends. How to cite this article: Zhang, X. et al. ARGONAUTE PIWI domain and microRNA duplex structure regulate small RNA sorting in Arabidopsis . Nat. Commun. 5:5468 doi: 10.1038/ncomms6468 (2014).